Mechanisms of charge transfer and redistribution in LaAlO3/SrTiO3revealed by high-energy optical conductivity In condensed matter physics the quasi two-dimensional electron gas at the interface of two different insulators, polar LaAlO 3 on nonpolar SrTiO 3 (LaAlO 3 /SrTiO 3 ) is a spectacular and surprising observation. This phenomenon is LaAlO 3 film thickness dependent and may be explained by the polarization catastrophe model, in which a charge transfer of 0.5 e − from the LaAlO 3 film into the LaAlO 3 /SrTiO 3 interface is expected. Here we show that in conducting samples (≥4 unit cells of LaAlO 3 ) there is indeed a ~0.5 e − transfer from LaAlO 3 into the LaAlO 3 /SrTiO 3 interface by studying the optical conductivity in a broad energy range (0.5–35 eV). Surprisingly, in insulating samples (≤3 unit cells of LaAlO 3 ) a redistribution of charges within the polar LaAlO 3 sublayers (from AlO 2 to LaO) as large as ~0.5 e − is observed, with no charge transfer into the interface. Hence, our results reveal the different mechanisms for the polarization catastrophe compensation in insulating and conducting LaAlO 3 /SrTiO 3 interfaces. Some of the most exciting condensed matter physics problems are found at the interfaces of dissimilar materials [1] . The behaviour of electrons at these interfaces would be governed by electronic reconstruction mechanisms [2] leading to a variety of exotic quantum phenomena [1] . In conjunction with X-ray and electron spectroscopy techniques [3] , [4] , [5] , [6] , [7] with their inherent advantages and constraints, an experimental technique that can directly reveal hidden quantum phenomena at buried interfaces is highly desirable. In this paper we demonstrate the potency of high-energy optical reflectivity coupled with spectroscopic ellipsometry and study an interface consisting of two dissimilar insulators: polar LaAlO 3 and nonpolar SrTiO 3 revealing the details of the charge (electron) transfer among and within the layers that govern the conductivity of the buried interface. The quasi two-dimensional electron gas (2DEG) at the the buried interface of two different insulator oxides heterostructure, polar LaAlO 3 on nonpolar SrTiO 3 (LaAlO 3 /SrTiO 3 ) [8] has shown many interesting phenomena ranging from metal–insulator transition [9] , superconductivity [10] and magnetism [11] , [12] , [13] , [14] . According to the controversial but compelling polarization catastrophe model, the polar sublayers of LaAlO 3 ((LaO) + and (AlO 2 ) − ) give rise to a polarization field inside LaAlO 3 that causes an electronic potential build-up as the LaAlO 3 film thickness increases. To counter this, a charge transfer of 0.5 e − per unit cell (uc) (~3 × 10 14 cm −2 ) from LaAlO 3 into the LaAlO 3 /SrTiO 3 interface is required [15] , [16] . Various techniques have shown a charge transfer much less than this. For example, X-ray-based techniques [5] , [6] have estimated up to 1.1 × 10 14 cm −2 while transport measurements [9] , [10] , [11] yield substantially smaller number of carriers of ~10 13 cm −2 . It has been suggested that charge localization effects might limit the number of mobile charges that can be measured by transport [7] , [17] , and thus if a technique can measure and quantify both the localized and delocalized charges, one might be able to evaluate the actual charge transfer [5] , [6] , [7] . Another unresolved important issue is the insulating case of LaAlO 3 /SrTiO 3 (≤3 uc of LaAlO 3 ). Transport measurements [9] have shown that the conducting interface only exists above a certain critical thickness of LaAlO 3 , typically ≥4 uc (although cationic stoichiometry, for example the La/Al ratio of LaAlO 3 film, may also affect the interface conductivity, with conducting LaAlO 3 /SrTiO 3 observed to have slightly Al-rich LaAlO 3 film [18] ). This means that the charge transfer into the interface required for countering the polarization catastrophe does not happen when the thickness of LaAlO 3 is below 4 uc. According to the prevalent polarization catastrophe model, this means the polarization field should be present for ≤3 uc of LaAlO 3 . One way to verify the model is to measure this polarization potential build-up in insulating LaAlO 3 /SrTiO 3 , which is predicted to be 0.24 V Å −1 (or ~0.9 V per uc of LaAlO 3 ) [19] . However, attempts to measure this have not been successful using core-level X-ray photoemission spectroscopy (XPS) [20] , [21] , in which the measured core-level shift in LaAlO 3 is only ~0.1 eV per uc of LaAlO 3 , much less than expected. If the changes in the band structure are predominantly near the valence bands and the Fermi level, then the appropriate technique should directly probe states near the valence bands and the Fermi level. Let us approach the problem from a different angle. Another way to overcome the polarization potential is by charge redistribution within the LaAlO 3 layers. In a Gedankenexperiment , we hypothesize an extreme case of charge redistribution of 1 e − between the AlO 2 and LaO sublayers of LaAlO 3 , which is also adequate to compensate the polarization potential, although the actual amount of charge redistribution might be restricted by electrostatics. Hence, instead of measuring the potential build-up in the layers, one can measure the charge redistribution within the layers directly. This can be done by measuring the optical conductivity involving states below and above the valence bands, the conduction bands and the Fermi level, and then use the f-sum rule, which represents charge conservation, to quantify the charge redistribution. Furthermore, recent band structure calculations and surface X-ray diffraction measurements suggest that distortions of the LaAlO 3 lattice (buckling) may partly compensate the polarization field in insulating LaAlO 3 /SrTiO 3 (refs 22 , 23 , 24 , 25 ). Interestingly, when the interface becomes conducting at LaAlO 3 thickness ≥4 uc, this distortion decreases and ultimately vanishes [24] , [25] , indicating that the buckling mechanism is unique to the insulating case of LaAlO 3 /SrTiO 3 . This raises another important question: since the buckling is a structural change, will the electronic structure change appropriately, and manifest as a charge redistribution within the LaAlO 3 layer itself? Thus, it is again critical to be able to measure these intralayer charge redistributions. As mentioned earlier, a direct way to probe the electronic band structure and charge (localized and delocalized) redistribution mechanisms is to measure the complex dielectric response of the material from which the optical conductivity can be extracted in a broad energy range [26] , [27] , [28] . Here we use a combination of spectroscopic ellipsometry and ultraviolet–vacuum ultraviolet (UV-VUV) reflectivity to probe the intrinsic properties of the LaAlO 3 /SrTiO 3 interface using photon with energies between 0.5 and 35 eV. Owing to a stabilized Kramers–Kronig transformation [29] , [30] , the strength of this experimental approach allows one to measure the charge transfer of both delocalized and localized charges accurately using the optical f-sum rule. Since localized electrons are inaccessible to electrical transport measurements, but are accessible by photons, we overcome a severe constraint. In particular, the optical transitions involving AlO 2 sublayer of LaAlO 3 is very distinct and well separated from the ones involving LaO sublayer, so that the internal charge redistribution within the LaAlO 3 sublayers can be clearly identified. The same is also true for the TiO 2 and SrO sublayers of SrTiO 3 . Here we show that in conducting LaAlO 3 /SrTiO 3 (4 and 6 uc of LaAlO 3 film on SrTiO 3 ), there is indeed a charge transfer from LaAlO 3 into the interface, and that the amount of charge transfer is ~0.5 e − . In the insulating case (2 and 3 uc of LaAlO 3 film on SrTiO 3 ), we surprisingly observe ~0.5 e − charge redistribution from AlO 2 to LaO sublayers, within the LaAlO 3 layers. This suggests that for the insulating case the polarization catastrophe could be partly overcome by the above-mentioned charge redistribution, which may be a consequence of the buckling of the LaAlO 3 lattice. Structural and transport measurements LaAlO 3 /SrTiO 3 samples were prepared by growing LaAlO 3 film on top of TiO 2 -terminated (001) SrTiO 3 using pulsed laser deposition [12] . The atomic force microscopy (AFM) topography image of the TiO 2 -terminated SrTiO 3 substrate in Fig. 1a clearly shows the atomically flat surface with uc steps. Four high-quality samples with varying thickness of 2, 3, 4 and 6 uc of LaAlO 3 film were prepared as a model interface system for the high-energy optical studies. The growth of the films was monitored using reflective high-energy electron diffraction ( Fig. 1b ). After LaAlO 3 deposition, AFM topography measurements show that the atomically flat surface with uc step and terrace structure of SrTiO 3 is preserved, with surface roughness of ~1 Å (see Fig. 1c,d ). This ensures that surface roughness effects do not adversely affect the optical measurements. Transport measurements ( Fig. 1e ), which were taken before and after the optics measurements, show consistently that 2 and 3 uc samples are insulating with carrier density and conductivity below the measurement limit, while 4 and 6 uc ones are conducting with carrier density of 4–6 × 10 13 cm −2 and conductivity of 4–8 × 10 −5 Ω −1 , consistent with previous transport results [9] , [10] , [11] . 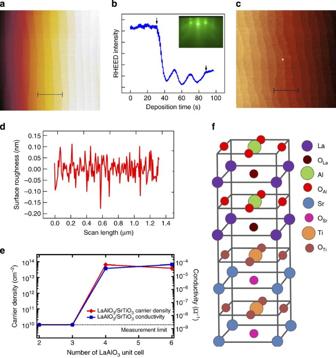Figure 1: Characterization results and crystal structure of LaAlO3/SrTiO3. (a) AFM topography image of TiO2-terminated SrTiO3substrate. Scale bar, 1 μm. (b) Reflective high-energy electron diffraction (RHEED) oscillations obtained for growth of 3 unit cells (uc) of LaAlO3film on SrTiO3substrate; inset shows obtained RHEED pattern after the LaAlO3growth. (c) AFM topography image of 4 uc LaAlO3/SrTiO3, showing the preserved atomically smooth surface. Scale bar, 1 μm. (d) The surface roughness of 4 uc LaAlO3/SrTiO3as extracted from the AFM data, measured to be ~1 Å. For other LaAlO3/SrTiO3samples (2, 3 and 6 uc LaAlO3/SrTiO3), the roughness variation and the surface AFM images are found to not alter very much as the LaAlO3thickness is below 15 uc and the layer-by-layer growth mode is preserved. (e) Electrical transport data of the LaAlO3/SrTiO3samples as a function of LaAlO3film thickness. (f) Crystal structure of LaAlO3/SrTiO3. Figure 1: Characterization results and crystal structure of LaAlO 3 /SrTiO 3 . ( a ) AFM topography image of TiO 2 -terminated SrTiO 3 substrate. Scale bar, 1 μm. ( b ) Reflective high-energy electron diffraction (RHEED) oscillations obtained for growth of 3 unit cells (uc) of LaAlO 3 film on SrTiO 3 substrate; inset shows obtained RHEED pattern after the LaAlO 3 growth. ( c ) AFM topography image of 4 uc LaAlO 3 /SrTiO 3 , showing the preserved atomically smooth surface. Scale bar, 1 μm. ( d ) The surface roughness of 4 uc LaAlO 3 /SrTiO 3 as extracted from the AFM data, measured to be ~1 Å. For other LaAlO 3 /SrTiO 3 samples (2, 3 and 6 uc LaAlO 3 /SrTiO 3 ), the roughness variation and the surface AFM images are found to not alter very much as the LaAlO 3 thickness is below 15 uc and the layer-by-layer growth mode is preserved. ( e ) Electrical transport data of the LaAlO 3 /SrTiO 3 samples as a function of LaAlO 3 film thickness. ( f ) Crystal structure of LaAlO 3 /SrTiO 3 . Full size image The perovskite LaAlO 3 uc ( Fig. 1f ) can be divided into two sublayers: LaO and AlO 2 , in which theoretical calculations have shown that the band structures of these discriminated sublayers are indeed different [19] , [22] , leading to distinct optical transitions. To accommodate the assignments of these optical transitions, we define O La as the O in the LaO plane and O Al as the O in the AlO 2 plane. Similarly, SrTiO 3 also has similar layered perovskite structure and thus can also be divided into two sublayers: SrO and TiO 2 . Then O Sr is defined as O that belongs to SrO sublayer, while O Ti is defined as the one in TiO 2 . Similarly, the O in the different planes of SrTiO 3 can also lead to distinct optical transitions. This discrimination is important, as discussed later, because it can reveal the intra- and interlayer charge transfer mechanism in LaAlO 3 /SrTiO 3 for both the insulating and conducting samples. Spectroscopic ellipsometry and high-energy reflectivity Our main observation is the high-energy reflectivity of LaAlO 3 /SrTiO 3 at different thicknesses of LaAlO 3 as compared with bulk LaAlO 3 and SrTiO 3 as shown in Fig. 2a . Note that, because of the challenge in making optical measurements over such a broad energy range, in this study we have only measured a selected set of samples as representative of insulating (2 and 3 uc) and conducting (4 and 6 uc) LaAlO 3 /SrTiO 3 . Thus, further measurements on a larger set of samples may be important in further deepening our analyses. It can be seen that the reflectivity spectra of the insulating 2 and 3 uc LaAlO 3 /SrTiO 3 are similar, and the same is true for the conducting 4 and 6 uc LaAlO 3 /SrTiO 3 . Surprisingly, there are huge differences between reflectivity of insulating and conducting samples. These differences occur more significantly at high photon energies, particularly in the energy ranges of 9–14 eV and 14–21 eV. In the 9–14-eV range, the reflectivity of conducting samples is lower than insulating samples, while in the 14–21-eV range the opposite occurs. In contrast, between 4 and 9 eV, the differences are less, and below 4 eV they are negligible. This signifies why going beyond conventional (up to ~5 eV) spectroscopic ellipsometry is important. (Note that the spectroscopic ellipsometry data are crucial for the normalization of the derived dielectric functions from the reflectivity measurements made up to 35 eV as shown in Supplementary Methods .) The electronic band structures of the insulating and conducting LaAlO 3 /SrTiO 3 are very different at high energy, and these differences are critical in revealing the true nature of LaAlO 3 /SrTiO 3 interface. Furthermore, since reflectivity and spectroscopic ellipsometry are sensitive to unpercolated clusters of charges [31] , the similarity of the reflectivity of insulating 2 and 3 uc LaAlO 3 /SrTiO 3 also implies that there is no evidence of precursor of percolation effects in the insulating samples, especially the 3 uc LaAlO 3 /SrTiO 3 (ref. 32 ). 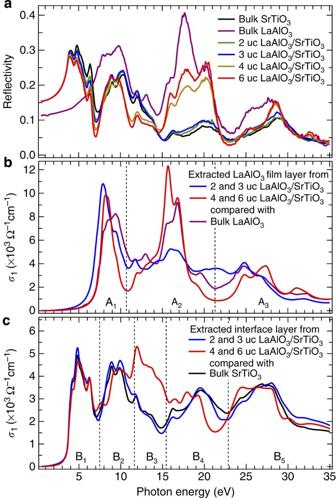Figure 2: Reflectivity and optical conductivity of each layer of LaAlO3/SrTiO3. (a) Reflectivity of LaAlO3/SrTiO3as compared with bulk LaAlO3and bulk SrTiO3. (b) Extracted optical conductivity (σ1) of LaAlO3films at different thickness of LaAlO3film, compared with bulk LaAlO3. (c) Extracted optical conductivity of the LaAlO3/SrTiO3interface at different thickness of LaAlO3film, compared with bulk SrTiO3. Note that the plots for 2 and 3 unit cells (uc) LaAlO3/SrTiO3are the same because of the nature of the iteration analysis used to extractσ1from reflectivity, and the same is true for the 4 and 6 uc LaAlO3/SrTiO3. Theσ1plots are divided into several energy regions, A1–A3for LaAlO3and B1–B5for SrTiO3and the interface. The regions are defined based on the distinct optical transitions associated with it, which in turn is based on theoretical calculations and previous reflectivity and valence electron energy loss spectroscopy36,37,38,39,40. Figure 2: Reflectivity and optical conductivity of each layer of LaAlO 3 /SrTiO 3 . ( a ) Reflectivity of LaAlO 3 /SrTiO 3 as compared with bulk LaAlO 3 and bulk SrTiO 3 . ( b ) Extracted optical conductivity ( σ 1 ) of LaAlO 3 films at different thickness of LaAlO 3 film, compared with bulk LaAlO 3 . ( c ) Extracted optical conductivity of the LaAlO 3 /SrTiO 3 interface at different thickness of LaAlO 3 film, compared with bulk SrTiO 3 . Note that the plots for 2 and 3 unit cells (uc) LaAlO 3 /SrTiO 3 are the same because of the nature of the iteration analysis used to extract σ 1 from reflectivity, and the same is true for the 4 and 6 uc LaAlO 3 /SrTiO 3 . The σ 1 plots are divided into several energy regions, A 1 –A 3 for LaAlO 3 and B 1 –B 5 for SrTiO 3 and the interface. The regions are defined based on the distinct optical transitions associated with it, which in turn is based on theoretical calculations and previous reflectivity and valence electron energy loss spectroscopy [36] , [37] , [38] , [39] , [40] . Full size image For detailed analysis, we turn our discussion to optical conductivity, σ 1 , because it fulfils the optical f-sum rule, which is related to number of charges excited by the photons. For bulk materials like bulk LaAlO 3 and bulk SrTiO 3 , σ 1 can be extracted directly from reflectivity using the Kramers–Kronig analysis [29] , [30] . On the other hand, LaAlO 3 /SrTiO 3 is layered along the <001> direction (perpendicular to the (001) surface of the sample) owing to its heterostructure nature as well as the presence of the conducting layer at LaAlO 3 /SrTiO 3 interface. For this reason, the reflectivity of LaAlO 3 /SrTiO 3 is analysed based on standard theory of wave propagation in a stratified media [33] , [34] . The analysis naturally leads to a three-layered structure for the conducting LaAlO 3 /SrTiO 3 : LaAlO 3 film layer on top, bulk SrTiO 3 substrate at the bottom and an interface layer sandwiched in between, representing the 2DEG of the conducting samples. A self-consistent iteration procedure is used to extract the thickness and dielectric function of each layer, and as long as the iteration is convergent, the starting assumption of these parameters should have little effect, if any, on the final obtained values (see Supplementary Methods for details). From the analysis, it is found that the thickness of this interface layer is ~5 nm, consistent with previous observation using hard XPS [5] , cross-sectional conducting tip AFM [35] and the upper limit for the superconducting layer thickness of LaAlO 3 /SrTiO 3 (ref. 10 ). This result also suggests that the high-energy reflectivity can be used to measure the thickness of interface layer. For insulating LaAlO 3 /SrTiO 3 , the analysis naturally converges into an effective two-layered structure instead. This means for insulating LaAlO 3 /SrTiO 3 the σ 1 at interface is very similar to that of bulk SrTiO 3 as discussed later. This can be easily understood owing to the absence of the conducting interface layer. Now, σ 1 of each individual layer can be extracted separately, so that we can analyse the concomitant evolution of each individual layer of LaAlO 3 /SrTiO 3 as the interface changes from insulating to conducting. Spectra of σ 1 for each layer are shown in Fig. 2b,c . It should be noted that the plots for 2 and 3 uc LaAlO 3 /SrTiO 3 are the same owing to the nature of the iteration process (see Supplementary Methods ), and the same is true for the 4 and 6 uc LaAlO 3 /SrTiO 3 . For LaAlO 3 , one can, based on band structure calculations [36] , [37] , divide σ 1 into three main optical regions, while σ 1 of SrTiO 3 can be divided into five main optical regions [38] , [39] , [40] . Every transition is unique and originates from different orbitals in each layer and sublayer, and these are summarized in Table 1 . Furthermore, the polarization of the incident light is also taken into account in assigning the optical transitions. Since the incident light is linearly polarized parallel to the sample surface, the majority of the optical transitions occur in the in-plane direction within each sublayer, allowing us to study spectral weight transfers between the different sublayers. For example, in A 1 region of LaAlO 3 , the transition is from O La -2 p to La-4 d , 5 f , both of which reside within the LaO sublayer of LaAlO 3 . The other transitions also follow this convention. Table 1 Main optical transitions of bulk LaAlO 3 and bulk SrTiO 3 . Full size table Figure 2b shows that σ 1 of LaAlO 3 film of insulating and conducting LaAlO 3 /SrTiO 3 is dramatically different as compared with bulk LaAlO 3 . Particularly, σ 1 in A 1 region of LaAlO 3 film in the insulating samples is higher than the bulk value, while for the conducting samples it is lower. Meanwhile, the reverse is true in A 2 region. It is very clear that there are spectral weight transfers occurring between these three regions when the thickness of LaAlO 3 film increases and the interface goes from insulating to conducting state. It can be seen ( Fig. 2c ) that σ 1 of the interface layer to a significant extent resembles σ 1 of the bulk SrTiO 3 . This indicates that the electronic interface layer is SrTiO 3 -like, and that the conducting layer mostly resides in SrTiO 3 side rather than LaAlO 3 . The most significant change in σ 1 happens at B 3 region when the interface becomes conducting. In bulk SrTiO 3 , that region corresponds to a valley with no main optical transition. Interestingly, for the conducting samples a completely new peak emerges in that region. This implies that when the interface becomes conducting, a new characteristic interface state emerges representing the presence of the 2DEG. According to previous reports [3] , [4] , [5] , [6] , [7] , [17] , [19] , [22] , the 2DEG resides in the Ti-3 d -t 2g state of SrTiO 3 , so this new interface state should also have Ti-3 d -t 2g characteristic. Thus, based on the optical selection rules, the optical transition at B 3 region may be assigned to originate from this new interface state to unoccupied states of higher O orbitals (see Table 1 ). One should note that the σ 1 spectra of the interface layer of conducting LaAlO 3 /SrTiO 3 does not show Drude response, consistent with previous infrared spectroscopic ellipsometry experiment [41] . The σ 1 analysis is very important because it can be linked to the effective number of electrons associated with a particular optical transition, N , using partial f-sum rule, where e is the elementary charge, m is the electron mass and V is the unit volume. The E 1 and E 2 indicate the energy boundaries of that particular transition in the σ 1 plot. We then define n eff as the N of each layer relative to either bulk LaAlO 3 (for LaAlO 3 film) or bulk SrTiO 3 (for interface layer) values. The advantage of this definition is that any changes in N in LaAlO 3 film or the interface layer can be distinguished from the bulk properties. In LaAlO 3 /SrTiO 3 (and thin films in general), the thickness of the LaAlO 3 film and interface layer is finite, so n eff distributes over this finite thickness. If we assume that the distribution is uniform over each uc, the n eff per uc, n uc , can be defined such that where d is the thickness in uc. In this case, the unit volume V becomes the volume occupied by each sublayer (LaO and AlO 2 for LaAlO 3 and SrO and TiO 2 for SrTiO 3 ), so that the unit of n uc is the number of charge per sublayer. Thus, n eff , which is the total amount of charge redistribution and transfer corresponding to a particular optical transition, can be obtained by integrating n uc over the layer thickness, as shown in Fig. 3 . (The procedure to obtain n eff is further explained in Methods). 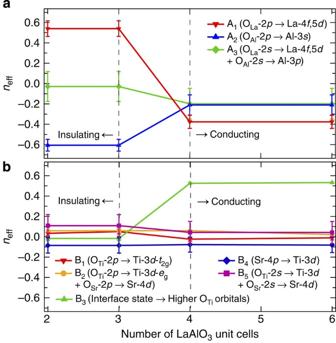Figure 3: The amount of charge redistribution and transfer in insulating and conducting LaAlO3/SrTiO3. (a) The amount of charge redistribution and transfer corresponding to different energy regions in theσ1plots of the LaAlO3film layer, relative to bulk LaAlO3values and plotted against LaAlO3film thickness. (b) The amount of charge redistribution and transfer corresponding to different energy regions in theσ1plots of the LaAlO3/SrTiO3interface layer, relative to bulk SrTiO3values and plotted against LaAlO3film thickness. Each of these energy regions can be attributed to distinct optical transitions36,37,38,39,40. The error bars are obtained from the resolution limitation of the optics measurements and the errors introduced during the reflectivity normalization procedure. Figure 3: The amount of charge redistribution and transfer in insulating and conducting LaAlO 3 /SrTiO 3 . ( a ) The amount of charge redistribution and transfer corresponding to different energy regions in the σ 1 plots of the LaAlO 3 film layer, relative to bulk LaAlO 3 values and plotted against LaAlO 3 film thickness. ( b ) The amount of charge redistribution and transfer corresponding to different energy regions in the σ 1 plots of the LaAlO 3 /SrTiO 3 interface layer, relative to bulk SrTiO 3 values and plotted against LaAlO 3 film thickness. Each of these energy regions can be attributed to distinct optical transitions [36] , [37] , [38] , [39] , [40] . The error bars are obtained from the resolution limitation of the optics measurements and the errors introduced during the reflectivity normalization procedure. Full size image We start our discussion with insulating samples. As shown in Fig. 3a , n eff of A 1 region of LaAlO 3 film increases by ~0.5 e − , while for A 2 region it decreases, also by ~0.5 e − . The net amount of the charge transfer in LaAlO 3 film is thus (+0.5 e − )+(−0.5 e − )=0. This indicates a redistribution of ~0.5 e − from O Al -2 p (AlO 2 sublayer) to O La -2 p (LaO sublayer), as shown in Table 1 . On the basis of f-sum rule, this directly implies that there is no net charge transfer into the LaAlO 3 /SrTiO 3 interface. As a result, the LaAlO 3 /SrTiO 3 interface remains insulating. Since the LaAlO 3 film (and the system as a whole) remains insulating, the ~0.5 e − charge redistribution does not result in the creation of electrons and holes in the LaO and AlO 2 sublayers but rather an increase of covalence between the LaO and AlO 2 sublayers, leading to the measured charge redistribution. One way to interpret these data is by considering that the charge redistribution is uniform for all LaAlO 3 layers. In this case, the covalence of AlO 2 becomes modified from −1 to −(1− n uc ) and the covalence of LaO from +1 to +(1− n uc ) ( Fig. 4a ). The n uc is ~0.25 e − −0.3 e − for the 2 uc LaAlO 3 /SrTiO 3 , and ~0.17 e − −0.2 e − for the 3 uc LaAlO 3 /SrTiO 3 (see Methods). This charge redistribution within the LaAlO 3 sublayers (electronic reconstruction [2] ) can thus help to decrease the potential build-up in the LaAlO 3 film and partially compensate the polarization catastrophe. Combined with ionic reconstruction mechanisms such as the buckling and ionic relaxations effects predicted [22] , [23] and observed earlier using surface X-ray diffraction [24] , [25] and second harmonic generation [32] , what we are measuring in terms of charge redistribution may arise from such a mechanism. 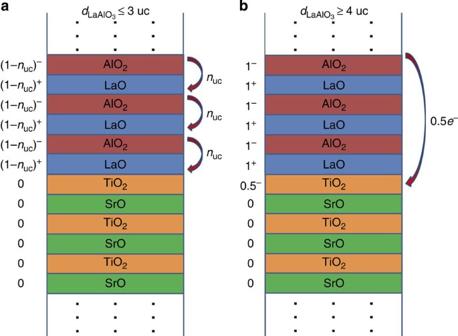Figure 4: Simplified pictorial layer-resolved electronic configuration model of LaAlO3/SrTiO3. (a) Layer-resolved electronic configuration model of insulating LaAlO3/SrTiO3, showing the charge redistribution from AlO2sublayer into LaO sublayer if the redistribution is assumed to be uniform across the LaAlO3film. Thenucis ~0.25e−−0.3e−for the 2 uc LaAlO3/SrTiO3and ~0.17e−−0.2e−for the 3 uc LaAlO3/SrTiO3. The charge redistribution can partially counteract the potential build-up due to polarization catastrophe15,16and keep the system insulating. (b) Layer-resolved electronic configuration model of conducting LaAlO3/SrTiO3, showing the overall charge transfer of 0.5e−from LaAlO3film into the LaAlO3/SrTiO3interface, consistent with the polarization catastrophe model. In this simple picture, the extra 0.5e−is depicted to reside only within the first uc of interface, while in our results it is distributed over the ~5 nm thickness on the interface. To ensure charge conservation, one of the upper layers of LaAlO3(that is, in the dot-signed region above the depicted third layer of LaAlO3) should have AlO2sublayer with valence state of (AlO2)0.5−instead of (AlO2)−. Figure 4: Simplified pictorial layer-resolved electronic configuration model of LaAlO 3 /SrTiO 3 . ( a ) Layer-resolved electronic configuration model of insulating LaAlO 3 /SrTiO 3 , showing the charge redistribution from AlO 2 sublayer into LaO sublayer if the redistribution is assumed to be uniform across the LaAlO 3 film. The n uc is ~0.25 e − −0.3 e − for the 2 uc LaAlO 3 /SrTiO 3 and ~0.17 e − −0.2 e − for the 3 uc LaAlO 3 /SrTiO 3 . The charge redistribution can partially counteract the potential build-up due to polarization catastrophe [15] , [16] and keep the system insulating. ( b ) Layer-resolved electronic configuration model of conducting LaAlO 3 /SrTiO 3 , showing the overall charge transfer of 0.5 e − from LaAlO 3 film into the LaAlO 3 /SrTiO 3 interface, consistent with the polarization catastrophe model. In this simple picture, the extra 0.5 e − is depicted to reside only within the first uc of interface, while in our results it is distributed over the ~5 nm thickness on the interface. To ensure charge conservation, one of the upper layers of LaAlO 3 (that is, in the dot-signed region above the depicted third layer of LaAlO 3 ) should have AlO 2 sublayer with valence state of (AlO 2 ) 0.5− instead of (AlO 2 ) − . Full size image Another possible scenario that can be considered to interpret the data is that, instead of involving the whole LaAlO 3 layers, the charge redistribution only happens at the topmost (that is, surface) LaAlO 3 layer. In this case, the covalence of surface AlO 2 becomes modified from −1 to −0.5 and the covalence of surface LaO from +1 to +0.5, but the deeper LaAlO 3 layer remains unchanged, since the charge redistribution is confined only in the surface (that is, surface reconstruction). In this scenario, the surface charge redistribution is still able to partially compensate the polarization catastrophe, but it is in less of an agreement with the buckling effects, since the buckling was observed experimentally, and supported by theoretical calculations [22] , [23] , [24] , [25] , to affect the whole LaAlO 3 film, and not only the surface. On the other hand, for conducting samples we observe a different phenomenon. The n eff of both A 1 and A 2 regions of LaAlO 3 film decreases ( Fig. 3a ). For A 1 region it decreases by ~0.3 e − −0.4 e − , while for A 2 region it decreases by ~0.2 e − , leading to an overall ~0.5 e − decrease of n eff in the LaAlO 3 film. At the same time, for the interface layer the most significant change that happens when LaAlO 3 /SrTiO 3 becomes conducting is the increase of n eff of B 3 region by ~0.5 e − ( Fig. 3b ). The total charge transfer within the whole LaAlO 3 /SrTiO 3 sample is thus again 0, with the decrease of ~0.5 e − in LaAlO 3 film compensated by the increase of ~0.5 e − at the interface. On the basis of f-sum rule, this clearly indicates that there is a charge transfer of ~0.5 e − from the LaAlO 3 film into the interface to form the 2DEG ( Fig. 4b ), consistent with the polarization catastrophe model [15] , [16] . On the basis of the definition of n eff , this ~0.5 e − extra charge at the interface is distributed over the ~5 nm thickness of the interface (which mostly resides in the SrTiO 3 side). Moreover, it can be seen from Fig. 2c that the B 3 peak, which involves the transition from the new interface state that contains this ~0.5 e − extra charge, is very broad (~4 eV wide), which means that the ~0.5 e − is distributed over a rather wide energy range. This may be one of the reasons why transport experiments can only measure a fraction of this ~0.5 e − , since only a small portion of the charge is delocalized and thus able to contribute to electrical conductivity. Furthermore, Fig. 3b also shows that the n eff of B 1 and B 5 regions, both of which involve transitions into the unoccupied Ti-3 d -t 2g states, decrease by ~0.05 e − (that is, ~10% of 0.5 e − ). This implies that the new interface state of conducting LaAlO 3 /SrTiO 3 has Ti-3 d -t 2g characteristic [3] , [4] , [5] , [6] , [7] , [17] , [19] , [22] , so the extra ~0.5 e − also partially fills the previously unoccupied Ti-3 d -t 2g state of SrTiO 3 . This decrease is consistent with previous observations using X-ray absorption spectroscopy experiments [3] , [6] . In X-ray absorption spectroscopy at Ti- L 3,2 edges of conducting LaAlO 3 /SrTiO 3 , the excitation to the unoccupied Ti-3 d -t 2g states also decreases compared with bulk SrTiO 3 . Intriguingly, these decreases are much smaller if one assumes that all of the ~0.5 e − extra charge partially fills the Ti-3 d -t 2g -unoccupied density of state (DOS). This is because, based on this assumption, one would expect to observe the decrease of Ti-3 d -t 2g -unoccupied DOS (and thus the n eff of B 1 and B 5 regions) in conducting LaAlO 3 /SrTiO 3 also by an equivalent of ~0.5 e − . However, this is not the case, which implies that the ~0.5 e − extra charge contained within the new interface state does not only reduce the number of unoccupied Ti-3 d DOS, but surprisingly also other states at even higher energies, implying the importance of strong correlations and hybridizations effects in explaining the interlayer charge transfer in conducting LaAlO 3 /SrTiO 3 (refs 26 , 42 , 43 ). Another interesting observation to note is that in the conducting samples, the n eff of A 3 region of LaAlO 3 film also decreases by ~0.2 e − . The transition in this region corresponds to O-2 s state, which is strongly localized and directly corresponds to the availability of oxygen in the LaAlO 3 film. Thus, the decrease of O-2 s DOS can indicate the presence of oxygen vacancies in the LaAlO 3 film of the conducting samples. For 4 uc LaAlO 3 /SrTiO 3 , there are 24 e − in O-2 s state of LaAlO 3 ; thus, the ~0.2 e − decrease is equivalent to ~1% oxygen vacancy. This is interesting because it has been suggested that the presence of oxygen vacancies in LaAlO 3 film may enhance the charge transfer from LaAlO 3 film into LaAlO 3 /SrTiO 3 interface [7] , [44] , [45] . Because of the charge transfer into the interface, the LaAlO 3 film lacks ~0.5 e − (that is, has additional ~0.5 holes), so the extra e − created by the oxygen vacancy may partially compensate these holes and stabilize the charge transfer. Interestingly, in insulating LaAlO 3 /SrTiO 3 , this oxygen vacancies signature is not observed. It is noteworthy to reconcile our results with photoconductivity effects observed in LaAlO 3 /SrTiO 3 . Previous transport results [46] , [47] have shown that when LaAlO 3 /SrTiO 3 was illuminated by photons with energies higher than the SrTiO 3 bandgap, its conductivity could increase because of the presence of photo-generated carriers. On the basis of hard XPS data [5] , the amount of these photo-generated carriers is estimated to be 2.1 × 10 13 cm −2 (~0.03 e − ), which is much smaller than the number of e − contributed to the charge transfer and charge redistributions observed in our results (~0.5 e − ). Thus, the photoconductivity effects might only influence the estimated n eff by ~6%, and do not affect our analysis adversely. Recent observations have also indicated that the cationic stoichiometry, for example, the La/Al ratio in LaAlO 3 film, may affect the electrical properties of LaAlO 3 /SrTiO 3 (refs 18 , 48 , 49 ). How this cationic stoichiometric effects would influence the high-energy optical conductivity of insulating and conducting LaAlO 3 /SrTiO 3 is an important open question. Thus, its interplay with the charge transfer and redistribution phenomena as observed in high-energy optical conductivity still remains to be answered. In summary, we have shown that high-energy reflectivity and spectroscopic ellipsometry studies of LaAlO 3 /SrTiO 3 have revealed significant differences between the charge redistribution of insulating (2 and 3 uc of LaAlO 3 ) and charge transfer mechanisms of conducting (4 and 6 uc of LaAlO 3 ) LaAlO 3 /SrTiO 3 . In insulating LaAlO 3 /SrTiO 3 , ~0.5 e − charge redistribution is observed between the AlO 2 and LaO sublayers and partially compensates the polarization catastrophe. In the conducting samples, ~0.5 e − is measured to be transferred from LaAlO 3 film into the interface, which is consistent with the polarization catastrophe model. We believe that this study reveals the nature of the intra- and interlayer charge redistributions and charge transfers in LaAlO 3 /SrTiO 3 , and hence opens a path to understand the various electronic reconstructions involving the interfaces of complex oxides heterostructures. Furthermore, the use of high-energy reflectivity coupled with spectroscopic ellipsometry could be extended to other similar polar and nonpolar oxide interface systems. Sample preparation LaAlO 3 /SrTiO 3 samples were prepared by growing LaAlO 3 film on top of (001) SrTiO 3 substrates obtained from Crystec using pulsed laser deposition [12] . Before the growth, the SrTiO 3 substrates were treated using HF and are annealed at 950 °C for 2 h in O 2 flow to achieve the desired TiO 2 surface termination [50] . The AFM topography image of the TiO 2 -terminated SrTiO 3 substrate in Fig. 1a clearly shows the atomically flat surface with uc steps. The growth target was LaAlO 3 single crystal, also obtained from Crystec. The deposition pressure was 10 −3 Torr, with background pressure of 10 −9 Torr. The deposition temperature was 750 °C, with cooling rate of 10 °C min −1 at the deposition pressure. The laser pulse frequency was 1 Hz. Four samples with varying thickness of 2, 3, 4 and 6 uc of LaAlO 3 film were made, as monitored using reflective high-energy electron diffraction ( Fig. 1b ). After LaAlO 3 deposition, AFM topography measurements show that the atomically flat surface with uc step and terrace structure of SrTiO 3 is preserved, with surface roughness of ~1 Å (see Fig. 1c,d ). Optics measurements The optical conductivity were obtained using a combination of spectroscopic ellipsometry (0.5–5.6 eV) and UV–VUV reflectivity (3.7–35 eV) measurements [26] , [27] , [28] . The details of the optical measurements are as follow. The spectroscopic ellipsometry measurements were performed in the spectral range between 0.5 and 5.6 eV by using an SE 850 ellipsometer at room temperature [51] . Three different incident angles of 60°, 70° and 80° from the sample normal were used, and the incident light was 45° linearly polarized from the plane of incident. For reflectivity measurements in the high-energy range between 3.7 and 35 eV, we used the SUPERLUMI beamline at the DORIS storage ring of HASYLAB (DESY) [52] . The incoming photon was incident at the angle of 17.5° from the sample normal with linear polarization parallel to the sample surface. The sample chamber was outfitted with a gold mesh to measure the incident photon flux after the slit of the monochromator. The measurements were performed in ultrahigh vacuum environment (chamber pressure of 5 × 10 −10 mbar) at room temperature. before these measurements, the samples were heated up to 400 K in ultrahigh vacuum to ensure that there was no additional adsorbate layers on the surface of the samples. The obtained UV–VUV reflectivity data were calibrated by comparing it with the luminescence yield of sodium salicylate (NaC 7 H 5 O 3 ) and the gold mesh current. These as-measured UV–VUV reflectivity data were further normalized by using the self-normalized reflectivity extracted from spectroscopic ellipsometry [34] , [51] , and the two normalized data were appended to obtain the combined reflectivity from 0.5 to 35 eV (see Supplementary Fig. 1 ). Analysis of optics data Both the spectroscopic ellipsometry and the combined reflectivity data were analysed using a combination of the Drude–Lorentz oscillator multilayer fitting [33] , [34] and self-consistent iteration method (see Supplementary Methods ). Owing to its multilayered nature, the LaAlO 3 /SrTiO 3 samples, especially the conducting cases, are considered to have the following three layers: the LaAlO 3 film on top, the SrTiO 3 substrate at the bottom and the interface layer in between (see Supplementary Fig. 2 ), consistent with previous observation using cross-sectional conducting tip AFM [35] . Since the spectroscopic ellipsometry data were taken at three different incident angles of 60°, 70° and 80°, it was fitted using angle-dependent iteration method (see Supplementary Methods ), and the fitting results are shown in Supplementary Figs 3, 4, 5, 6 and 7 . Supplementary Figure 4 also shows that the thickness of the conducting interface layer is ~5 nm, consistent with previous observations [5] , [10] , [35] . Furthermore, from these variable angle spectroscopic ellipsometry results, the absence of absorbate layer and the absence of significant anisotropy can also be inferred. On the other hand, the normalized UV–VUV reflectivity data were fitted using thickness-dependent iteration method (see Supplementary Methods ), and the results of the fitting are shown in Supplementary Fig. 8 . Complex dielectric function of LaAlO 3 /SrTiO 3 From the analysis described above, the complex dielectric function, ε ( ω ), of each layer of LaAlO 3 /SrTiO 3 can be extracted from the high-energy reflectivity of LaAlO 3 /SrTiO 3 ( Fig. 2a ), as presented in Fig. 5 . In turn, this ε ( ω ) can be converted into optical conductivity σ 1 using σ 1 ( ω )= ε 0 ε 2 ( ω ) ω , as presented in Fig. 2b,c . In Fig. 5a,b , it can be seen that the ε ( ω ) of the LaAlO 3 film layer for both insulating and conducting LaAlO 3 /SrTiO 3 is very different than that of bulk LaAlO 3 , which shows that the band structure of LaAlO 3 film is very different than bulk LaAlO 3 . Meanwhile, the ε ( ω ) at the interface of the insulating samples (2 and 3 uc LaAlO 3 /SrTiO 3 , see Fig. 5c ) is very similar to that of bulk SrTiO 3 , which can be explained by the absence of the 2DEG in the insulating samples. Interestingly, for the conducting samples (4 and 6 uc LaAlO 3 /SrTiO 3 , see Fig. 5d ) there are new features around 8–12 eV for ε 1 and 11–16 eV for ε 2 , which, on further analysis (see Discussions), are related to the presence of the conducting interface in those sample. 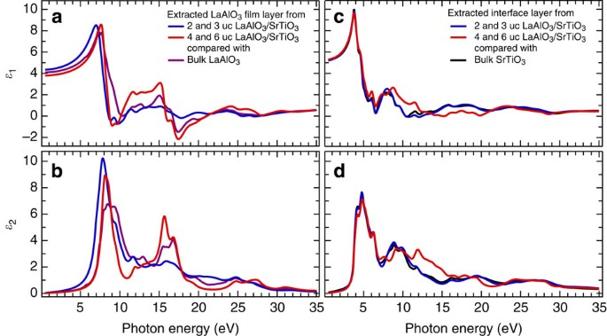Figure 5: Complex dielectric function of each layer of LaAlO3/SrTiO3. (a) Real part of complex dielectric function (ε1) of LaAlO3film, compared with bulk LaAlO3. (b) Imaginary part of complex dielectric function (ε2) of LaAlO3film, compared with bulk LaAlO3. (c) Theε1of LaAlO3/SrTiO3interface, compared with bulk SrTiO3. (d) Theε2of LaAlO3/SrTiO3interface, compared with bulk SrTiO3. Note that the plots for 2 and 3 unit cells (uc) are the same because of the nature of the thickness-dependent iteration, and the same is true for the 4 and 6 uc case. Figure 5: Complex dielectric function of each layer of LaAlO 3 /SrTiO 3 . ( a ) Real part of complex dielectric function ( ε 1 ) of LaAlO 3 film, compared with bulk LaAlO 3 . ( b ) Imaginary part of complex dielectric function ( ε 2 ) of LaAlO 3 film, compared with bulk LaAlO 3 . ( c ) The ε 1 of LaAlO 3 /SrTiO 3 interface, compared with bulk SrTiO 3 . ( d ) The ε 2 of LaAlO 3 /SrTiO 3 interface, compared with bulk SrTiO 3 . Note that the plots for 2 and 3 unit cells (uc) are the same because of the nature of the thickness-dependent iteration, and the same is true for the 4 and 6 uc case. Full size image Estimation of charge transfer and redistribution From equations (1) and (2), we can extract the n uc , which is the amount of charge redistribution and transfer per uc associated with a particular optical transition relative to the bulk values. To get the accurate number, we need to carefully consider within what volume V in the uc the electrons reside. Both LaAlO 3 and SrTiO 3 crystal structures can be thought of as an alternating layer structure. LaAlO 3 consists of alternating polar (LaO) + and (AlO 2 ) − sublayers, while SrTiO 3 consists of alternating nonpolar SrO and TiO 2 sublayers (see Figs 1d and 4 ). Owing to this layered structure, in a first approximation each cation (La and Al for LaAlO 3 , Sr and Ti for SrTiO 3 ) only occupies a volume of half uc (instead of the full one uc). For example, the La of LaAlO 3 has to share the space of one uc with Al (with each getting half), and similarly the Sr of SrTiO 3 has to share with Ti. Furthermore, for LaAlO 3 , the valence electrons of the O atoms that belong to the two different sublayers (LaO and AlO 2 ) contribute to two different optical transitions in the σ 1 spectra ( Fig. 2b and Table 1 ). For simplicity, O La is defined as the O in the LaO plane and O Al as the O in the AlO 2 plane. Thus, O La also has to share the space of one uc with O Al , with each getting the space of half uc. The same is true for SrTiO 3 , where the O Sr in the SrO plane also has to share the space of one uc with the O Ti in the TiO 2 plane. This implies that the valence electrons belonging to the different ions can also be approximated to reside in a volume of half uc. For this reason, to obtain the n uc the volume V is chosen to be the volume of half uc of LaAlO 3 (lattice constant a 0 =3.81 Å) or SrTiO 3 ( a 0 =3.905 Å), whichever applicable. This consideration makes the unit of n uc to be the number of charge per sublayer. The result for this n uc estimation is shown in Fig. 6 . For 2 uc LaAlO 3 /SrTiO 3 , the n uc is ~0.25 e − −0.3 e − , while for 3 uc LaAlO 3 /SrTiO 3 , the n uc is ~0.17 e − −0.2 e − . Then, the n eff , which is the total amount of charge redistribution and transfer corresponding to a particular optical transition can be obtained by integrating n uc over the layer thickness, as shown in Fig. 3 . 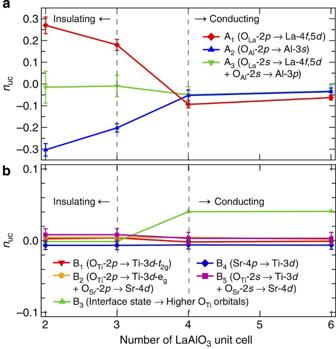Figure 6: Effective number of charge per unit cell (uc) of LaAlO3and interface layer of LaAlO3/SrTiO3. (a) The effective number of charge per uc,nuc, of LaAlO3film, if the charge distribution is assumed to be uniform over the LaAlO3thicknesses (2, 3, 4 and 6 uc). (b) Thenucof the LaAlO3/SrTiO3interface, if the charge distribution is assumed to be uniform over the interface thickness (~5.3 nm). Each of these energy regions can be attributed to distinct optical transitions36,37,38,39,40. The error bars are obtained from the resolution limitation of the optics measurements and the errors introduced during the reflectivity normalization procedure. Figure 6: Effective number of charge per unit cell (uc) of LaAlO 3 and interface layer of LaAlO 3 /SrTiO 3 . ( a ) The effective number of charge per uc, n uc , of LaAlO 3 film, if the charge distribution is assumed to be uniform over the LaAlO 3 thicknesses (2, 3, 4 and 6 uc). ( b ) The n uc of the LaAlO 3 /SrTiO 3 interface, if the charge distribution is assumed to be uniform over the interface thickness (~5.3 nm). Each of these energy regions can be attributed to distinct optical transitions [36] , [37] , [38] , [39] , [40] . The error bars are obtained from the resolution limitation of the optics measurements and the errors introduced during the reflectivity normalization procedure. Full size image The error bars in Figs 3 and 6 are estimated as follows. It is assumed that there are two main sources of random errors in the data: from the resolution limitation of the optics measurements (estimated to be ~2%) and from the errors introduced in the normalization process (estimated to be ~5%). These errors affect the reflectivity data (that is, Δ R ), and to obtain the corresponding errors for σ 1 (Δ σ ) and thus n eff , the errors are propagated using LaAlO 3 band structure calculation Unlike SrTiO 3 that has been studied very thoroughly [38] , [39] , [40] , previous reports that study the band structure and high photon-energy properties of LaAlO 3 in a detailed and comprehensive manner remain quite scarce [36] , [37] . Because of this, we performed our own band structure calculation of LaAlO 3 to complement those previous studies. The results can be used as a tool to determine the high photon-energy optical transition assignments of LaAlO 3 , as listed in Table 1 . The details of the calculation are as follows. Cubic LaAlO 3 has a space group of with an experimental lattice parameters of a = b = c =3.8106 Å at 821 K (ref. 53 ). The calculations were performed using CASTEP code [54] . Geometry optimization had been carried out with local density approximation functional using cutoff energy of 1,500 eV and a 15 × 15 × 15 Monkhorst–Pack grid [55] that corresponds to 120 k -points in the irreducible Brillouin zone. The cutoff energy and k -point mesh had been tested and converged to energy differences of 1 × 10 −5 and 4 × 10 −5 eV per atom, respectively. Ultrasoft pseudopotentials were generated ‘on the fly’ with valence states 4 f , 5 s , 5 p , 5 d , 6 s for La, 3 s , 3 p for Al and 2 s , 2 p for O. The electronic minimization method used for the self-consistent field calculation was density mixing [56] with a self-consistent field tolerance of 2.0 × 10 −6 eV per atom. The geometry optimization was carried out by the Broyden–Fletcher–Goldfarb–Shanno algorithm [57] with energy, force and displacement tolerances of 5.0 × 10 −6 eV per atom, 1.0 × 10 −2 eV Å −1 and 5.0 × 10 −4 Å, respectively. The optimized lattice parameter was found out to be 3.73 Å. Converged DOS calculation was carried out with a k -mesh of 20 × 20 × 20 and consistent with previous calculations [36] , [37] . The calculation results are displayed in Fig. 7 . 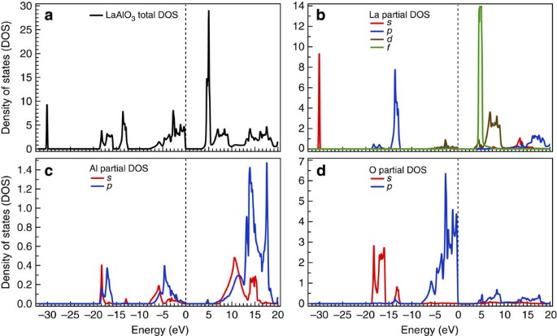Figure 7: Theoretical band structure of LaAlO3. (a) Total density of states (DOS) of LaAlO3. (b) Partial DOS of La. (c) Partial DOS Al. (d) Partial DOS of O. The dotted lines are the Fermi level. Figure 7: Theoretical band structure of LaAlO 3 . ( a ) Total density of states (DOS) of LaAlO 3 . ( b ) Partial DOS of La. ( c ) Partial DOS Al. ( d ) Partial DOS of O. The dotted lines are the Fermi level. Full size image How to cite this article: Asmara, T. C. et al. Mechanisms of charge transfer and redistribution in LaAlO 3 /SrTiO 3 revealed by high-energy optical conductivity. Nat. Commun. 5:3663 doi: 10.1038/ncomms4663 (2014).